ArhGAP30 promotes p53 acetylation and function in colorectal cancer Covalent modification adding acetyl groups to the C terminus of the p53 protein has been suggested to be required for its functional activation as a tumour suppressor. However, it remains largely unknown how p53 acetylation is deregulated in colorectal cancer (CRC), which is the third most commonly diagnosed cancer worldwide. Here we show that ArhGAP30, a Rho GTPase-activating protein, is a pivotal regulator for p53 acetylation and functional activation in CRC. ArhGAP30 binds to p53 C-terminal domain and P300, facilitating P300-mediated acetylation of p53 at lysine 382. ArhGAP30 expression is required for p53 activation upon DNA damage stress, and the level of ArhGAP30 correlates with p53 acetylation and functional activation in CRC tissues. Moreover, low level of ArhGAP30 expression associates with poor survival of CRC patients. In summary, ArhGAP30 is required for p53 acetylation and functional activation in CRC, and the expression of ArhGAP30 is a potential prognostic marker for CRC. The p53 tumour suppressor is a central node of a cellular stress response pathway that is crucial in suppressing cancer formation in many tissue and cell types [1] , [2] , [3] , [4] and in regulating other processes such as pigmentation, fecundity, cellular metabolism, mitochondrial respiration, stem cell maintenance and early embryonic development [5] , [6] , [7] , [8] , [9] . p53 is tightly regulated, such that it usually exists in a latent form, and at low levels, in unstressed cells. Upon cellular stresses such as DNA damage, replicative stress, oncogene activation and hypoxia, p53 is activated and initiates cellular responses such as DNA repair, cell cycle arrest, apoptosis, senescence and metabolic regulation [10] , [11] , [12] , [13] . p53 determines these cellular fates primarily through its ability to regulate the transcription of numerous target genes through direct, sequence-specific, DNA binding [14] , [15] . The p53 protein includes a transactivation domain (amino acids 1–44), a proline-rich domain (PRD; 64–92), a central DNA-binding domain (DBD; 102–292), a tetramerization domain (TD; 325–356) and a C-terminal domain (CTD; 357–393). The DBD is found to bind DNA in a sequence-dependent manner and can trigger apoptosis on the mitochondria [16] , and the PRD seems to be involved in the interaction with p300 (ref. 17 ). Nonetheless, the role of CTD is still elusive. Early studies suggested that the p53 CTD, whose interaction with DNA is not sequence dependent, acts as a negative regulator of the core DBD [18] . However, later reports concluded that p53 requires its CTD for efficient recognition of target gene sequences [19] . Although mice with C-terminal lysines mutated into arginines appeared similar to wild-type (WT) mice [20] , [21] , a more recent study found that mutant mice lacking p53 CTD caused an increase in p53 activity and phenotypes related to human telomere syndromes [22] . While no existing mechanistic model can perfectly explain all experimental observations, the p53 CTD is clearly required for proper functions of p53 (ref. 23 ). Although ubiquitin-mediated proteasomal degradation is well accepted as a key mechanism for regulation of p53 expression levels [24] , [25] , [26] , [27] , [28] , [29] , it is still elusive how p53 is activated. There have been conflicting results on the question of whether p53 post-translational modification (PTM), such as phosphorylation or acetylation, are essential or only play a subtle role in the p53 response. Recent studies by several groups have reported that acetylation is critically required for the activation of the p53 protein [30] , [31] , [32] , [33] . Acetylation of lysine residues in the C terminus of p53 has been found with important functional roles for the activation of this tumour suppressor protein [34] . In support of these, different factors have been reported to affect p53 acetylation under various physiological or pathological conditions, including the proteins ARF [35] , MOZ [36] , WTX [37] and nucleolar RNA [38] . However, it remains poorly understood how p53 acetylation is regulated in colorectal cancer (CRC), which is the third most commonly diagnosed cancer worldwide and caused 608,000 deaths in 2008 (ref. 39 ). In the present study, we report that ArhGAP30, a Rho GTPase-activating protein [40] , regulates p53 acetylation in a Rho-independent manner in CRC. First, we found significant downregulation of ArhGAP30 in CRC and its precancerous lesion, and further analysis identified significant association between ArhGAP30 downregulation and poor patient survival. Gene expression profiling study identified the p53 pathway as a major regulatory target of ArhGAP30. We acquired both in vitro and in vivo data supporting the regulatory effects of ArhGAP30 on p53 acetylation and functional activation. Interestingly, the effects of ArhGAP30 on p53 is independent of its function as a RhoGAP, but is mediated by interaction with the p300 acetyltransferase. These findings add to the complexity of p53 PTM that leads to its functional activation, and highlight ArhGAP30 as a potential prognostic factor in CRC. ArhGAP30 downregulation associates with CRC and poor outcome First, we analysed published microarray data sets and found significant downregulation of ArhGAP30 in CRC and its precancerous lesion, colorectal adenoma ( Supplementary Fig. 1 ). We further experimentally confirmed that ArhGAP30 mRNA and protein levels are significantly downregulated in CRC tissues than in normal colorectal tissues ( P <0.001, Student’s t -test; Fig. 1a,b ). 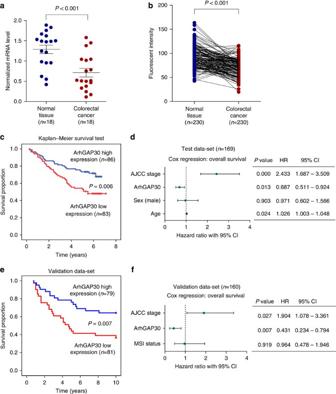Figure 1: Downregulation of ArhGAP30 in CRC and its association with poor survival. (a) ArhGAP30 mRNA expression level in normal (n=18) and CRC (n=18) tissues (P<0.001, Student’st-test). The values were determined by qRT–PCR and normalized by 18S rRNA (bars indicate means±s.d.). (b) Statistics of ArhGAP30 protein expression levels in CRC and paired normal tissues as determined by immunofluorescence. The results include 180 pairs from tissue microarrays and 50 pairs from Renji hospital (P<0.001, pairedt-test). (c) Kaplan–Meier plot of 169 patients with survival data (from tissue arrays) stratified by ArhGAP30 protein expression level. Patients expressing lower levels of ArhGAP30 (compared with average level in CRC) displayed shorter overall survival (54.5 months) than the other patients (47.5 months;P=0.006, Kaplan–Meier survival test). (d) Multivariate Cox regression model indicating the effects of different factors on CRC patient survival (n=169). ThePvalue, hazard ratio (HR) and 95% confidence interval (95% CI) have been shown for each factor. After adjustment for AJCC stage, sex and age, ArhGAP30 upregulation (compared with average level in CRC) still showed significant association with lower risk for mortality (P=0.013, 95% CI 0.511–0.924). (e) Kaplan–Meier survival analysis of an independent validation data set that included 160 Norwegian cases41. Upregulation of ArhGAP30 mRNA (compared with average level in CRC) associated with longer overall survival than the other patients (79.2 versus 96.0 months,P=0.007). (f) After adjustment for AJCC stage and microsatellite instability (MSI) status by Cox regression, ArhGAP30 upregulation (compared with average level in CRC) retained significant association with lower risk for mortality (P=0.007, 95% CI 0.234–0.794). We compared different clinicopathological features of CRC cases stratified by ArhGAP30 expression level, and found that ArhGAP30 downregulation significantly associated with larger tumour size (diameter>5 cm, P =0.04), advanced pathological stage ( P =0.003), Dukes stage ( P =0.028) and American Joint Committee on Cancer (AJCC) stage ( P =0.038, all comparisons by Fisher’s exact test; Supplementary Table 1 ). Downregulation of ArhGAP30 also associated with shorter overall survival (median survival 47.5 versus 54.5 months, 7-year follow-up, P =0.0065, Kaplan–Meier test; Fig. 1c ), and multivariate analysis correcting for age, sex and tumour stage confirmed this (hazard ratio 0.687, 95% confidence interval 0.511–0.924; P =0.013; Fig. 1d ). The association between ArhGAP30 and survival of CRC patients was validated using an independent data set that included Norwegian CRC cases with 10-year survival follow-up (GEO accession GSE24551; ref. 41 ). Notably, the overall survival of patients in the ArhGAP30 downregulation group was significantly shorter than in the upregulation group (79.2 versus 96.0 months, P =0.007; Fig. 1e ), and multivariate analysis suggested significant association after adjustment for tumour stage and microsatellite instability (MSI) status (hazard ratio 0.431, 95% confidence interval 0.234–0.794; P =0.007; Fig. 1f ). These results collectively suggest that ArhGAP30 may be involved in CRC. Figure 1: Downregulation of ArhGAP30 in CRC and its association with poor survival. ( a ) ArhGAP30 mRNA expression level in normal ( n =18) and CRC ( n =18) tissues ( P <0.001, Student’s t -test). The values were determined by qRT–PCR and normalized by 18S rRNA (bars indicate means±s.d.). ( b ) Statistics of ArhGAP30 protein expression levels in CRC and paired normal tissues as determined by immunofluorescence. The results include 180 pairs from tissue microarrays and 50 pairs from Renji hospital ( P <0.001, paired t -test). ( c ) Kaplan–Meier plot of 169 patients with survival data (from tissue arrays) stratified by ArhGAP30 protein expression level. Patients expressing lower levels of ArhGAP30 (compared with average level in CRC) displayed shorter overall survival (54.5 months) than the other patients (47.5 months; P =0.006, Kaplan–Meier survival test). ( d ) Multivariate Cox regression model indicating the effects of different factors on CRC patient survival ( n =169). The P value, hazard ratio (HR) and 95% confidence interval (95% CI) have been shown for each factor. After adjustment for AJCC stage, sex and age, ArhGAP30 upregulation (compared with average level in CRC) still showed significant association with lower risk for mortality ( P =0.013, 95% CI 0.511–0.924). ( e ) Kaplan–Meier survival analysis of an independent validation data set that included 160 Norwegian cases [41] . Upregulation of ArhGAP30 mRNA (compared with average level in CRC) associated with longer overall survival than the other patients (79.2 versus 96.0 months, P =0.007). ( f ) After adjustment for AJCC stage and microsatellite instability (MSI) status by Cox regression, ArhGAP30 upregulation (compared with average level in CRC) retained significant association with lower risk for mortality ( P =0.007, 95% CI 0.234–0.794). Full size image ArhGAP30 induces cell cycle arrest and apoptosis Western blot analysis showed significantly lower levels of ArhGAP30 expression in human CRC LoVo and HCT116 cells (both carrying WT p53) than in normal epithelium CRL1790 cells ( Supplementary Fig. 2a ). To test the potential effects of ArhGAP30 in CRC cells, LoVo and HCT116 cells stably transfected with ArhGAP30 or control vector (validation of expression shown in Supplementary Fig. 2b ). Both wound-healing assay and Transwell migration test reported significant effect of ArhGAP30 on suppressing cell migration and invasion ( Fig. 2b–d and Supplementary Fig. 2c ). In addition, ectopic expression of ArhGAP30 significantly decreased the proliferation rate of LoVo and HCT116 cells ( P <0.001; Fig. 2e,f and Supplementary Fig. 2d ). Flow cytometry assay (described in Supplementary methods ) revealed G2/M cell cycle arrest of ArhGAP30-expressing cells, concomitant with a decrease in S-phase ( Fig. 2g–j ). Consistently, phycoerythrin-conjugated Annexin V staining revealed significantly increased cell apoptosis upon ArhGAP30 expression ( Fig. 2k–m ). 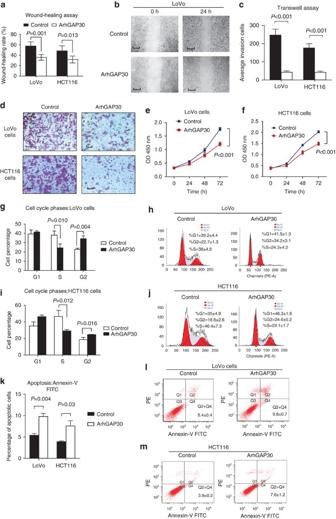Figure 2: ArhGAP30 suppresses invasion and induces apoptosis and cell cycle arrest of CRC cells. The LoVo and HCT116 cells were stably transfected with ArhGAP30 (LoVoArhGAP30and HCT116ArhGAP30) or control vector (LoVopcDNA3and HCT116pcDNA3) for subsequent analyses. Data in all statistical plots represent means±s.d. (n=4). (a) Statistical result of wound-healing rates for LoVoArhGAP30, HCT116ArhGAP30and control cell strains 24 h after treatment (Pvalues indicated, Student’st-test). (b) Representative images of wound-healing assay for LoVoArhGAP30and LoVopcDNA3cells. Scale bars, 200 μm. (c) Statistics of Transwell migration assay for LoVoArhGAP30and HCT116ArhGAP30lines compared with control lines 24 h after treatment. Results were based on four independent experiments (Student’st-test). (d) Representative images for Transwell migration assays. Cells that penetrated the filter were stained by Trypan blue, and images were acquired at the same magnitude. Scale bars,100 μm. (e,f) Proliferation of LoVoArhGAP30, HCT116ArhGAP30and control cells as determined by MTT assay. Thexaxis indicates the time after plating, and theyaxis presents the output of MTT assay (OD 450 nm). Results were based on four independent experiments. (g,h) Statistical results and representative images for the cell cycle phases of LoVoArhGAP30and LoVopcDNA3cells determined by Annexin V-labelled flow cytometry assay. Results were based on four independent experiments (Student’st-test). (i,j) Statistical results and representative images for cell cycle phases of HCT116ArhGAP30and HCT116pcDNA3cells determined by Annexin V-labelled flow cytometry assay. (k) Statistical results for the apoptosis of above cell strains as revealed by Annexin V-labelled flow cytometry assay. Results were based on four independent experiments (Student’st-test). (l,m) Fow cytometry using Annexin V suggested increased apoptosis of LoVoArhGAP30and HCT116ArhGAP30cells as compared with control cell lines (P=0.004 and 0.03, respectively, Student’st-test). (j) Representative images of Annexin V-labelled flow cytometry assays. FITC, fluorescein isothiocyanate. Figure 2: ArhGAP30 suppresses invasion and induces apoptosis and cell cycle arrest of CRC cells. The LoVo and HCT116 cells were stably transfected with ArhGAP30 (LoVo ArhGAP30 and HCT116 ArhGAP30 ) or control vector (LoVo pcDNA3 and HCT116 pcDNA3 ) for subsequent analyses. Data in all statistical plots represent means±s.d. ( n =4). ( a ) Statistical result of wound-healing rates for LoVo ArhGAP30 , HCT116 ArhGAP30 and control cell strains 24 h after treatment ( P values indicated, Student’s t -test). ( b ) Representative images of wound-healing assay for LoVo ArhGAP30 and LoVo pcDNA3 cells. Scale bars, 200 μm. ( c ) Statistics of Transwell migration assay for LoVo ArhGAP30 and HCT116 ArhGAP30 lines compared with control lines 24 h after treatment. Results were based on four independent experiments (Student’s t -test). ( d ) Representative images for Transwell migration assays. Cells that penetrated the filter were stained by Trypan blue, and images were acquired at the same magnitude. Scale bars,100 μm. ( e , f ) Proliferation of LoVo ArhGAP30 , HCT116 ArhGAP30 and control cells as determined by MTT assay. The x axis indicates the time after plating, and the y axis presents the output of MTT assay (OD 450 nm). Results were based on four independent experiments. ( g , h ) Statistical results and representative images for the cell cycle phases of LoVo ArhGAP30 and LoVo pcDNA3 cells determined by Annexin V-labelled flow cytometry assay. Results were based on four independent experiments (Student’s t -test). ( i , j ) Statistical results and representative images for cell cycle phases of HCT116 ArhGAP30 and HCT116 pcDNA3 cells determined by Annexin V-labelled flow cytometry assay. ( k ) Statistical results for the apoptosis of above cell strains as revealed by Annexin V-labelled flow cytometry assay. Results were based on four independent experiments (Student’s t -test). ( l , m ) Fow cytometry using Annexin V suggested increased apoptosis of LoVo ArhGAP30 and HCT116 ArhGAP30 cells as compared with control cell lines ( P =0.004 and 0.03, respectively, Student’s t -test). ( j ) Representative images of Annexin V-labelled flow cytometry assays. FITC, fluorescein isothiocyanate. Full size image Identification of p53-dependent effects of ArhGAP30 To probe the pathways regulated by ArhGAP30 on an unbiased basis, we performed gene expression profiling study on LoVo cells stably transfected with ArhGAP30 or control vector (Affymetrix HG-U133 Plus 2.0 array, data available on GEO: GSE49536). Assessment of Gene Ontology annotation revealed alterations in several pathways, including cell apoptosis ( n =63), cell cycle arrest ( n =29), cell migration ( n =18) and actin assembly ( n =8) ( Fig. 3a , detailed gene list in Supplementary Table 2 ). Notably, a considerable number of apoptotic (31/63) and cell cycle arresting (13/29) genes are well-established p53 downstream targets, including p21, CCNG1, PUMA, MDM2 , GADD45A and so on ( Fig. 3a ). Further, we analysed the occupancy of p53 on the promoters of ArhGAP3-induced genes using chromatin immunoprecipitation sequencing (ChIP-seq) data published previously [42] . Interestingly, 52% (409/781) of the ArhGAP30-induced genes had p53-bound regions near their transcription starting sites (TSSs), and this rate was significantly higher than the average p53 occupancy in the genome ( P <0.0001, χ 2 -test; Fig. 3b,c ). These findings suggest that ArhGAP30 may confer p53-dependent effects in CRCs. 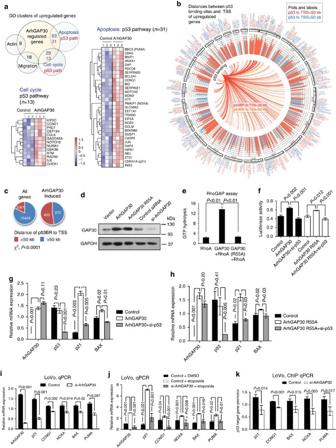Figure 3: p53-dependent but GAP-independent effects of ArhGAP30. (a) Affymetrix expression array identified ArhGAP30-regulated genes in different pathways. The Venn diagram indicates upregulated pathways, with p53-associated genes highlighted in red. The heat maps show cell cycle and apoptosis-related genes in the p53 pathway. (b) The Circos plot shows ArhGAP30-induced genes (histogram) that are either bound (in red) or not bound by p53 (in blue). The links in centre represent the binding of p53 to ArhGAP30-induced genes. When the distance between p53-binding region (p53BR) and gene transcription starting site (TSS) is <20 kb, the linked is shown in red. When the distance is between 20 and 50 kb, the link is in orange. (c) The pie plots show the number of genes bound by p53 (p53BR to TSS <50 kb) in the whole genome or in the set of ArhGAP30-induced genes. (d) Western blot showing the effective upregulation or silencing of ArhGAP30. (e) The RhoGAP assay showing the functions of ArhGAP30 and its R55A mutant on activating RhoA. Theyaxis indicates the level of GTP that is released by the hydrolysis reaction. Results were based on four independent experiments (Student’st-test, bars indicate means±s.d.). (f) The LoVo cells carrying WT p53 were transfected with PG13 reporter together with ArhGAP30 or its R55A mutant, in the absence or presence of specific siRNAs for p53. Theyaxis indicates luciferase activity as a ratio of firefly to renilla. Results were based on four independent experiments (Student’st-test, bars indicate means±s.d.). (g,h) The qRT–PCR assay measuring the levels of p53 downstream targets in LoVo cells expressing ectopic ArhGAP30 (g) or R55A mutant (h), in the absence or presence of p53 siRNAs. Results were based on four independent experiments (Student’st-test, bars indicate means±s.d.). (i) qRT-PCR showing the effects of ArhGAP30 silencing on expression of p53 target genes (bars indicate means±s.d.,n=4, Student’st-test). (j) Twenty-four hours after transfection with ArhGAP30 siRNAs or control siRNAs, cells were incubated with 20 μM etoposide for 5 h and analysed for the expression of indicated genes by qRT–PCR (bars indicate means±s.d.,n=4, Student’st-test). (k) LoVo cells were treated by ArhGAP30 siRNAs or control siRNAs, and the binding of p53 to target promoters was detected by ChIP coupled by qPCR (bars indicate means±s.d.,n=4, Student’st-test). Figure 3: p53-dependent but GAP-independent effects of ArhGAP30. ( a ) Affymetrix expression array identified ArhGAP30-regulated genes in different pathways. The Venn diagram indicates upregulated pathways, with p53-associated genes highlighted in red. The heat maps show cell cycle and apoptosis-related genes in the p53 pathway. ( b ) The Circos plot shows ArhGAP30-induced genes (histogram) that are either bound (in red) or not bound by p53 (in blue). The links in centre represent the binding of p53 to ArhGAP30-induced genes. When the distance between p53-binding region (p53BR) and gene transcription starting site (TSS) is <20 kb, the linked is shown in red. When the distance is between 20 and 50 kb, the link is in orange. ( c ) The pie plots show the number of genes bound by p53 (p53BR to TSS <50 kb) in the whole genome or in the set of ArhGAP30-induced genes. ( d ) Western blot showing the effective upregulation or silencing of ArhGAP30. ( e ) The RhoGAP assay showing the functions of ArhGAP30 and its R55A mutant on activating RhoA. The y axis indicates the level of GTP that is released by the hydrolysis reaction. Results were based on four independent experiments (Student’s t -test, bars indicate means±s.d.). ( f ) The LoVo cells carrying WT p53 were transfected with PG13 reporter together with ArhGAP30 or its R55A mutant, in the absence or presence of specific siRNAs for p53. The y axis indicates luciferase activity as a ratio of firefly to renilla. Results were based on four independent experiments (Student’s t -test, bars indicate means±s.d.). ( g , h ) The qRT–PCR assay measuring the levels of p53 downstream targets in LoVo cells expressing ectopic ArhGAP30 ( g ) or R55A mutant ( h ), in the absence or presence of p53 siRNAs. Results were based on four independent experiments (Student’s t -test, bars indicate means±s.d.). ( i ) qRT-PCR showing the effects of ArhGAP30 silencing on expression of p53 target genes (bars indicate means±s.d., n =4, Student’s t -test). ( j ) Twenty-four hours after transfection with ArhGAP30 siRNAs or control siRNAs, cells were incubated with 20 μM etoposide for 5 h and analysed for the expression of indicated genes by qRT–PCR (bars indicate means±s.d., n =4, Student’s t -test). ( k ) LoVo cells were treated by ArhGAP30 siRNAs or control siRNAs, and the binding of p53 to target promoters was detected by ChIP coupled by qPCR (bars indicate means±s.d., n =4, Student’s t -test). Full size image We manipulated ArhGAP30 expression in CRC cells ( Fig. 3d , full-length blots in Supplementary Fig. 3a ) and detected its effects on p53 transcriptional activity using luciferase reporter and quantitative reverse transcription (qRT–PCR) assays. We have also included a GAP-deficient mutant (R55A) as control, which is devoid of the catalytic arginine and thus loses its RhoGAP activity ( Fig. 3e ). Ectopic expression of ArhGAP30 significantly increased the transactivity of p53 on PG13 luciferase reporter that contained p53-responsive promoter sequence ( Fig. 3f ). Such effect was retained by the GAP-deficient R55A mutant, but knockdown of p53 blocked this effect in luciferase assay ( Fig. 3f ). In the qRT-PCR assay, ectopic expression of ArhGAP30 significantly increased the transactivation of a panel of p53 target genes including CDKN1A (p21), CCNG1, NOXA, BAX and PUMA ( Supplementary Fig. 3b,c ). The GAP-deficient R55A mutant retained this ability, but silencing p53 suppressed the effects of ArhGAP30 ( Fig. 3g,h ). These findings suggest significant p53-dependent but GAP-independent effects of ArhGAP30 on cell cycle and apoptosis-related genes. ArhGAP30 promotes p53 function upon DNA damage In both LoVo and HCT116 cells, knockdown of ArhGAP30 decreased the transactivation of p53 downstream target genes ( Fig. 3i and Supplementary Fig. 3d ). Further, we tested whether ArhGAP30 is required for the activation of p53 function in response to DNA damage stress. Exposure of LoVo and HCT116 cells to 20 μM etoposide induced substantial upregulation of p53 target genes CDKN1A , CCNG1 , NOXA , BAX and PUMA , but knockdown of ArhGAP30 by specific small-interfering RNAs (siRNAs) suppressed the transactivation of these genes (qRT–PCR data shown in Fig. 3j and Supplementary Fig. 3e ). The requirement of ArhGAP30 for p53 activation upon DNA damage was also confirmed by western blot ( Supplementary Fig. 3f ). In support to the role of ArhGAP30’s effects on p53 function, we found significant correlation between the expression of ArhGAP30 and p53 target genes, such as p21 , MDM2 , NOXA and so on ( Supplementary Fig. 3g ), according to the microarray data of The Cancer Genomic Atlas CRC cohort [43] . Further, we went to analyse whether ArhGAP30 affects the binding of p53 to target promoters in vivo by quantitative ChIP assay. To this end, LoVo cells that bear WT p53 were transfected with siRNAs specific for ArhGAP30 and treated with 20 μM etoposide, followed by ChIP using antibodies specific for p53. The DNA recovered by ChIP was specifically amplified for the promoter regions of target genes CDKN1A, CCGN1, BAX, NOXA and PUMA using qPCR. As a result, knockdown of ArhGAP30 significantly decreased the binding of p53 to target promoters ( Fig. 3k ). These data collectively demonstrate the requirement of ArhGAP30 for p53 activation, and provide mechanistic explanation for the effects of ArhGAP30 on cell cycle arrest and apoptosis. Dependence of ArhGAP30 effects on cell growth and migration Since ArhGAP30 has been found to affect actin dynamics and cell adhesion [40] , we tested whether the RhoGAP function of ArhGAP30 may cause its effects on cell cycle arrest and apoptosis. To this end, both LoVo and HCT116 cells were stably transfected with control vector, ArhGAP30 or the GAP-deficient R55A mutant, followed by detection by cell proliferation, apoptosis and migration assays. Intriguingly, the R55A mutant could still suppress cell proliferation ( Fig. 4a,b ), promote apoptosis ( Fig. 4c,d and Supplementary Fig. 4 ) and inhibit cell migration ( Fig. 4e,f ). However in p53-null HCT116 cells, ArhGAP30 and its R55A mutant failed to induce the expression of p21, BAX, PUMA and so on ( Fig. 4g–i ), and showed no significant effect on cell proliferation and apoptosis ( Fig. 4j–l ). These results consistently suggest that ArhGAP30 affect cell proliferation and apoptosis by p53-dependent mechanisms. 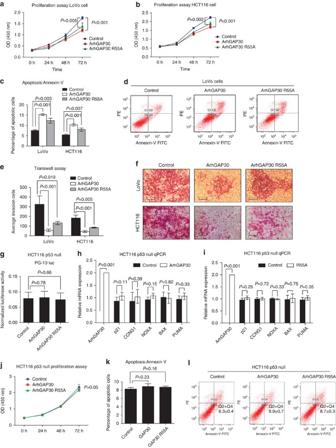Figure 4: Effects of ArhGAP30 on cell growth and migration are p53 dependent. (a,b) Proliferation of LoVo (a) and HCT116 cells (b) expressing ArhGAP30, the R55A mutant or control vector as detected by MTT assay. Thexaxis indicates time after plating, and theyaxis presents the readout of MTT assay (OD 450 nm). Results were based on four independent experiments (Student’st-test, bars indicate means±s.d.). (c) Statistical analysis on the apoptosis of LoVo and HCT116 cells expressing ArhGAP30, R55A mutant or control vector, based on Annexin V staining flow cytometry assay (bars indicate means±s.d.,n=4, Student’st-test). (d) Representative image for Annexin V staining flow cytometry assay of LoVo cells treated as described above. (e) Statistical results for the Transwell assay of above-described cells (bars indicate means±s.d.,n=4, Student’st-test). (f) Representative Transwell image of the indicated cells. Scale bars, 200 μm. (g) The HCT116 (p53-null) cells were transfected with PG13 reporter together with ArhGAP30 or its R55A mutant, followed by luciferase assay (bars indicate means±s.d.,n=4, Student’st-test). (h,i) qRT-PCR assay showing the effects of ArhGAP30 (h) and its R55A mutant (i) on the expression of p53 target genes (bars indicate means±s.d.,n=4, Student’st-test). (j) Effects of ArhGAP30 and its R55A mutant on the proliferation of HCT116 (p53-null) cells (bars indicate means±s.d.,n=4, Student’st-test). (k,l) Statistical result (k) and representative images (l) for the apoptosis of HCT116 (p53-null) cells as revealed by Annexin V staining flow cytometry assays (bars indicate means±s.d.,n=4, Student’st-test). FITC, fluorescein isothiocyanate. Figure 4: Effects of ArhGAP30 on cell growth and migration are p53 dependent. ( a , b ) Proliferation of LoVo ( a ) and HCT116 cells ( b ) expressing ArhGAP30, the R55A mutant or control vector as detected by MTT assay. The x axis indicates time after plating, and the y axis presents the readout of MTT assay (OD 450 nm). Results were based on four independent experiments (Student’s t -test, bars indicate means±s.d.). ( c ) Statistical analysis on the apoptosis of LoVo and HCT116 cells expressing ArhGAP30, R55A mutant or control vector, based on Annexin V staining flow cytometry assay (bars indicate means±s.d., n =4, Student’s t -test). ( d ) Representative image for Annexin V staining flow cytometry assay of LoVo cells treated as described above. ( e ) Statistical results for the Transwell assay of above-described cells (bars indicate means±s.d., n =4, Student’s t -test). ( f ) Representative Transwell image of the indicated cells. Scale bars, 200 μm. ( g ) The HCT116 (p53-null) cells were transfected with PG13 reporter together with ArhGAP30 or its R55A mutant, followed by luciferase assay (bars indicate means±s.d., n =4, Student’s t -test). ( h , i ) qRT-PCR assay showing the effects of ArhGAP30 ( h ) and its R55A mutant ( i ) on the expression of p53 target genes (bars indicate means±s.d., n =4, Student’s t -test). ( j ) Effects of ArhGAP30 and its R55A mutant on the proliferation of HCT116 (p53-null) cells (bars indicate means±s.d., n =4, Student’s t -test). ( k , l ) Statistical result ( k ) and representative images ( l ) for the apoptosis of HCT116 (p53-null) cells as revealed by Annexin V staining flow cytometry assays (bars indicate means±s.d., n =4, Student’s t -test). FITC, fluorescein isothiocyanate. Full size image ArhGAP30 enhances p53 acetylation in a p300-dependent manner Interestingly, we found that ectopic expression of ArhGAP30 enhanced the acetylation of p53 protein at Lys382 site ( Fig. 5a and Supplementary Fig. 5a ), which is a well-established PTM that activates p53 function [44] . The concomitant upregulation of p21 confirmed p53 activation ( Fig. 5a ). In addition, the GAP-deficient mutant R55A retained the ability to promote p53 acetylation ( Fig. 5a ). Consistently, knockdown of ArhGAP30 caused marked decrease in p53 Lys382 acetylation and p21 expression ( Fig. 5a ). When the acetylation site on position 382 was disrupted by a mutation (K382A), the effect of ArhGAP30 on p53 function was blocked. However, mutation of another potential acetylation position (K373A) did not affect the effect of ArhGAP30 ( Fig. 5b ), suggesting K382 as the key regulatory site of ArhGAP30. 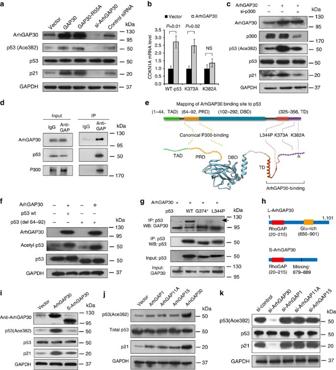Figure 5: ArhGAP30 binds p53 and promotes its acetylation by p300. (a) Western blot (WB) showing the levels of p53 Lys382 acetylation and p21 expression in LoVo cells transfected with ArhGAP30, the R55A mutant or specific siRNAs for ArhGAP30. GAPDH and ArhGAP30 were also detected as control. (b) The WT p53 or its mutants K373A or K382A was transfected to HCT116 (p53-null) cells together with ArhGAP30 or control vector, followed by qRT-PCR assay detecting the expression of CDKN1A (bars indicate means±s.d.,n=4, Student’st-test). (c) LoVo cells were transfected with ArhGAP30 plasmid in the absence or presence of siRNAs for p300. The levels of ArhGAP30, p300, Ace-p53 and p21 were detected by WB. (d) Specific antibody for ArhGAP30 was used to precipitate ArhGAP30 from LoVo cells, and the amounts of p53 and p300 in the precipitated complex were detected by WB. The input amounts of ArhGAP30, p53 and P300 are also detected as control. (e) Schematic representation for the structural domains of p53 protein. The p53 protein contains transactivation domain (TAD), PRD, DBD, TD and the extreme C-terminal region (in purple). Positions of the L344P, K373A and K382A mutations have been labelled in the graph. (f) WB showing the effect of ArhGAP30 on the acetylation of p53 devoid of its PRD (del 64–92). GAPDH was also detected as loading control. (g) Co-immunoprecipitation assay showing the interaction between ArhGAP30 and p53 G374stop (C-terminal-truncated) and L344P (tetramerization-disrupting) mutations. Both mutants were found to disrupt the interaction between ArhGAP30-p53. The black arrow indicates the band corresponding to ArhGAP30. (h) Structural domains of L-ArhGAP30 and S-ArhGAP30. The common RhoGAP domain is shown in red, and the Glu-rich domain unique for L-ArhGAP30 is shown orange. (i) WB showing the effects of L-ArhGAP30 and S-ArhGAP30 on p53 acetylation and p21 expression. Cells transfected with L-ArhGAP30 or S-ArhGAP30, and WB was used to analyse the expression of indicated proteins 48 h after transfection. (j) LoVo cells were transfected with ArhGAP1, ArhGAP11A, ArhGAP15 or ArhGAP30, and the levels of Ace-p53, total p53 and p21 were analysed by WB 48 h after transfection. (k) Specific siRNAs for ArhGAP30, ArhGAP, ArhGAP11A or ArhGAP15 were used to knockdown the indicated RhoGAPs, and the levels of Ace-p53, total p53 and p21 were analysed by WB. Figure 5: ArhGAP30 binds p53 and promotes its acetylation by p300. ( a ) Western blot (WB) showing the levels of p53 Lys382 acetylation and p21 expression in LoVo cells transfected with ArhGAP30, the R55A mutant or specific siRNAs for ArhGAP30. GAPDH and ArhGAP30 were also detected as control. ( b ) The WT p53 or its mutants K373A or K382A was transfected to HCT116 (p53-null) cells together with ArhGAP30 or control vector, followed by qRT-PCR assay detecting the expression of CDKN1A (bars indicate means±s.d., n =4, Student’s t -test). ( c ) LoVo cells were transfected with ArhGAP30 plasmid in the absence or presence of siRNAs for p300. The levels of ArhGAP30, p300, Ace-p53 and p21 were detected by WB. ( d ) Specific antibody for ArhGAP30 was used to precipitate ArhGAP30 from LoVo cells, and the amounts of p53 and p300 in the precipitated complex were detected by WB. The input amounts of ArhGAP30, p53 and P300 are also detected as control. ( e ) Schematic representation for the structural domains of p53 protein. The p53 protein contains transactivation domain (TAD), PRD, DBD, TD and the extreme C-terminal region (in purple). Positions of the L344P, K373A and K382A mutations have been labelled in the graph. ( f ) WB showing the effect of ArhGAP30 on the acetylation of p53 devoid of its PRD (del 64–92). GAPDH was also detected as loading control. ( g ) Co-immunoprecipitation assay showing the interaction between ArhGAP30 and p53 G374stop (C-terminal-truncated) and L344P (tetramerization-disrupting) mutations. Both mutants were found to disrupt the interaction between ArhGAP30-p53. The black arrow indicates the band corresponding to ArhGAP30. ( h ) Structural domains of L-ArhGAP30 and S-ArhGAP30. The common RhoGAP domain is shown in red, and the Glu-rich domain unique for L-ArhGAP30 is shown orange. ( i ) WB showing the effects of L-ArhGAP30 and S-ArhGAP30 on p53 acetylation and p21 expression. Cells transfected with L-ArhGAP30 or S-ArhGAP30, and WB was used to analyse the expression of indicated proteins 48 h after transfection. ( j ) LoVo cells were transfected with ArhGAP1, ArhGAP11A, ArhGAP15 or ArhGAP30, and the levels of Ace-p53, total p53 and p21 were analysed by WB 48 h after transfection. ( k ) Specific siRNAs for ArhGAP30, ArhGAP, ArhGAP11A or ArhGAP15 were used to knockdown the indicated RhoGAPs, and the levels of Ace-p53, total p53 and p21 were analysed by WB. Full size image Since the acetyltransferase CBP/p300 has been implicated in the acetylation of p53 protein [45] , we tested whether ArhGAP30 promoted p53 acetylation in a p300-dependent manner. In fact, knockdown of p300 abolished the effect of ArhGAP30 on p53 acetylation and p21 activation, thus confirmed the involvement of p300 ( Fig. 5c ). Moreover, extensive colocalization was found between ArhGAP30, p53 and P300 in the nucleus of cells that were exposed to DNA damage stress ( Supplementary Fig. 5b ), suggesting potential interaction between the three proteins. Consistently, pull down of ArhGAP30 resulted in the co-immunoprecipitation of both p53 and p300 ( Fig. 5d ), thus confirmed the complex formation by the three proteins. Further, we identified the regions of p53 that bind to ArhGAP30. When the proline-rich region (PRD, shown in Fig. 5e ) of p53 was deleted by mutation, ArhGAP30 could still promote p53 acetylation ( Fig. 5f ). However, the mutations that disrupted tetramerization (L344P) [46] or deleted the extreme C-terminal region of p53 (G374stop) were both able to abolish the p53–ArhGAP30 interaction ( Fig. 5g ). Thus, the TD and extreme C-terminal region of p53 are both required for binding to ArhGAP30. Predominant effect of ArhGAP30 full-length variant ArhGAP30 has been shown to have a full-length and a shorter splice variant, namely L-ARHGAP30 and S-ARHGAP30, respectively [40] . L-ARHGAP30 encodes a deduced 1,101-amino acid protein with an N-terminal GAP domain, followed by a proline-rich motif, a glutamic acid-rich motif and a second proline-rich motif near the C terminus. S-ARHGAP30 encodes a deduced 890-amino acid protein that lacks the glutamic acid-rich motif (shown in Fig. 5h ). We overexpressed L-ArhGAP30, S-ArhGAP30 and control vector in CRC cells, and detected acetylated p53 by western blot. Unlike L-ArhGAP30, the S-ArhGAP30 variant showed no effect on p53 acetylation ( Fig. 5i , also shown below). Of note, ArhGAP30 is predominantly expressed as the full-length (L-ArhGAP30) variant in CRC cells, and the band corresponding to S-ArhGAP30 is not detectable. Since the S-ArhGAP30 variant only differs from L-ArhGAP30 by the Glu-rich domain (679–889), it is very likely that the unique Glu-rich domain of ArhGAP30 is required for the effect on p53 acetylation. We have found previously that some RhoGAPs (for example, ArhGAP15, ArhGAP11A and ArhGAP1) can bind to and stabilize the p53 TD [47] . Since p53 is active in tetrameric conformation, these interactions lead to enhanced p53 activity. More specifically, we found that ectopic overexpression of ArhGAP15 could enhance p53 transactivity in CRC cells. However, here we show by western blot that overexpression of ArhGAP15, ArhGAP1 and ArhGAP1 could not affect p53 acetylation ( Fig. 5j ). The effect of ArhGAP30 on p21 expression (acetylation-based p53 activation) was much stronger than the other RhoGAPs (tetramerization based). In HCT116 CRC cells, knockdown of ArhGAP30 but not other RhoGAPs significantly decreased p53 acetylation and p21 expression ( Fig. 5k and Supplementary Fig. 5c ). The above findings consistently suggest that ArhGP30 has an outstanding role in p53 acetylation in CRC cells, thus providing an explanation for its strong prognostic effect in CRC. ArhGAP30 promotes p53 acetylation in vivo To test whether ArhGAP30 has a role in p53 acetylation in vivo in human CRC tissues, we evaluated the correlation between ArhGAP30 expression level and the extent of p53 acetylation at Lys382 by immunofluorescence ( Fig. 6a,b ). Notably, a significant correlation was found between ArhGAP30 expression and p53 Lys382 acetylation (Pearson correlation R =0.6177, P <0.0001; Fig. 6c ). When the CRC tissues were stratified by the expression level of ArhGAP30, a significant higher fraction of copy number variation in the genome was found in CRC tissues expressing lower levels of ArhGAP30 ( P =0.0012; Fig. 6d ). Since previous studies have found that mutant p53 can also be acetylated [35] , ArhGAP30 may have a stronger effect in tumours bearing WT p53. To test the prognostic effect of ArhGAP30 in CRCs with different p53 status, we analysed a microarray data set (GSE39582) that includes information for ArhGAP30 expression, TP53 gene status and patient survival. Interestingly, low expression of ArhGAP30 significantly associated with shorter survival in tumours carrying WT p53 but not mutant p53 ( Supplementary Fig. 6a,b ). These findings are consistent with the role of ArhGAP30 in p53 acetylation and activation in human CRC tissues. 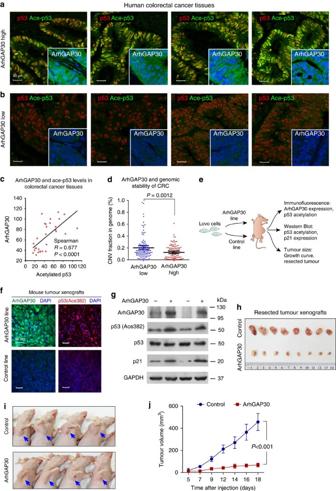Figure 6: ArhGAP30 regulates p53 acetylation and activationin vivo. (a,b) Human CRC tissues were immunostained for acetylated p53 at Lys382 (ace-p53, labelled in green), total p53 (in red) and ArhGAP30 (lower right quadrant, in green). Scale bars, 30 μm. Intensive p53 acetylation can be detected in CRC tissues expressing higher level of ArhGAP30 (a) but not in ArhGAP30-depleted CRC tissues (b). (c) Statistics of tissue immunofluorescence showing strong correlation between the levels of ArhGAP30 and acetylated p53 (n=29, Spearman correlationR=0.677,P<0.0001). (d) The fraction of genome with copy number variation (CNV) was significantly higher in CRC tissues expressing lower level of ArhGAP30. CRC tissues in The Cancer Genomic Atlas were stratified by ArhGAP30 expression levels (below or above median value in CRC), and the fraction of CNV in genome was compared between two groups (n=222, Mann–Whitney test,P=0.0012). (e) Schematic diagram illustrating the procedures forin vivotumour xenograft experiment. The LoVo cells stably expressing ArhGAP30 or pcDNA3 vector were, respectively, injected subcutaneously to nude mice to allow tumour formation, followed by the indicated analyses. (f) Immunofluorescence showing significant increase of acetylated p53 (labelled in red) in LoVoArhGAP30xenograft tumours. Scale bars, 50 μm. (g) Western blot confirmed the upregulation of acetylated p53 and p21 in LoVoArhGAP30xenograft tumours. GAPDH was detected as control. (h) Comparison of excised tumours sizes at the last time point. (i) Observed xenograft tumour sizes in LoVoArhGAP30and LoVopcDNA3groups (labelled by blue arrows). (j) The growth curves of LoVoArhGAP30and LoVopcDNA3xenograft tumours. A plateau was reached by LoVoArhGAP302 weeks after tumour seeding. The tumour sizes at the last time point was significantly smaller in LoVoArhGAP30group than in LoVopcDNA3group (P<0.001, Student’st-test, bars indicate means±s.d.n=8). Figure 6: ArhGAP30 regulates p53 acetylation and activation in vivo . ( a , b ) Human CRC tissues were immunostained for acetylated p53 at Lys382 (ace-p53, labelled in green), total p53 (in red) and ArhGAP30 (lower right quadrant, in green). Scale bars, 30 μm. Intensive p53 acetylation can be detected in CRC tissues expressing higher level of ArhGAP30 ( a ) but not in ArhGAP30-depleted CRC tissues ( b ). ( c ) Statistics of tissue immunofluorescence showing strong correlation between the levels of ArhGAP30 and acetylated p53 ( n =29, Spearman correlation R =0.677, P <0.0001). ( d ) The fraction of genome with copy number variation (CNV) was significantly higher in CRC tissues expressing lower level of ArhGAP30. CRC tissues in The Cancer Genomic Atlas were stratified by ArhGAP30 expression levels (below or above median value in CRC), and the fraction of CNV in genome was compared between two groups ( n =222, Mann–Whitney test, P =0.0012). ( e ) Schematic diagram illustrating the procedures for in vivo tumour xenograft experiment. The LoVo cells stably expressing ArhGAP30 or pcDNA3 vector were, respectively, injected subcutaneously to nude mice to allow tumour formation, followed by the indicated analyses. ( f ) Immunofluorescence showing significant increase of acetylated p53 (labelled in red) in LoVo ArhGAP30 xenograft tumours. Scale bars, 50 μm. ( g ) Western blot confirmed the upregulation of acetylated p53 and p21 in LoVo ArhGAP30 xenograft tumours. GAPDH was detected as control. ( h ) Comparison of excised tumours sizes at the last time point. ( i ) Observed xenograft tumour sizes in LoVo ArhGAP30 and LoVo pcDNA3 groups (labelled by blue arrows). ( j ) The growth curves of LoVo ArhGAP30 and LoVo pcDNA3 xenograft tumours. A plateau was reached by LoVo ArhGAP30 2 weeks after tumour seeding. The tumour sizes at the last time point was significantly smaller in LoVo ArhGAP30 group than in LoVo pcDNA3 group ( P <0.001, Student’s t -test, bars indicate means±s.d. n =8). Full size image To further evaluate the effect of ArhGAP30 on reactivating p53 in vivo , we established xenograft tumour models as described in Fig. 5e . The LoVo cells stably expressing ArhGAP30 (LoVo ArhGAP30 ) or control vector (LoVo pcDNA ) were, respectively, implanted subcutaneously into athymic nude mice to allow tumour formation, and tumour diameters were measured every 2 days. As a result, increased level of p53 Lys382 acetylation was found in LoVo ArhGAP30 xenograft tumours than in LoVo pcDNA tumours ( Fig. 5f ), concomitant with the upregulation of p21 in these tissues ( Fig. 5g ). The rescue of ArhGAP30 markedly reduced tumour size (by ~90%; Fig. 5h,i ), and a plateau phase was reached by the LoVo ArhGAP30 tumours 2 weeks after injection ( Fig. 5j ). These results suggest potential therapeutic value of ArhGAP30 rescue in p53 reactivation and tumour suppression in CRC. ArhGAP30 is a direct transcriptional target of p53 In both LoVo and HCT116 cells, we found that ArhGAP30 expression could be substantially induced by DNA damage ( Fig. 7a and Supplementary Fig. 7a ). We further detected ArhGAP30 expression level at different time points after etoposide treatment, and found that the upregulation of ArhGAP30 occurred after that of p53 ( Fig. 7b ). In fact ArhGAP30 displayed similar kinetics as p21, a well-established downstream target of p53 ( Fig. 7b ). By analysing the ArhGAP30 promoter sequence using the PROMO algorithm [48] , we found multiple putative p53-binding sequences near the TSS of ArhGAP30 (−217 to +97, shown in Fig. 7c ). We cloned this promoter sequence into a luciferase reporter vector and tested its response to p53. Importantly, p53 transactivated the intact ArhGAP30 promoter but not the mutated promoter sequence that was deleted for the putative p53-binding sites ( Fig. 7d ). To test the binding of p53 to ArhGAP30 promoter in vivo, we performed ChIP assay using a specific antibody for p53. Notably, the promoter region of ArhGAP30 was amplifiable from the DNA recovered from the immunoprecipitation complex ( Fig. 7e ). Further ChIP qPCR assay on LoVo cells overexpressing p53 also confirmed the recruitment of p53 to the promoter of ArhGAP30 ( Fig. 7f ). Ectopic expression of p53 significantly increased the expression of ArhGAP30 ( Fig. 7g ), while knockdown of ArhGAP30 blocked p53 acetylation and its transcriptional function on target genes p21, CCNG1, BAX, PUMA and NOXA ( Fig. 7h,i ). Thus, ArhGAP30 seems to function as both a downstream target and a upstream regulator of p53, constituting a positive feedback loop for p53 activation. 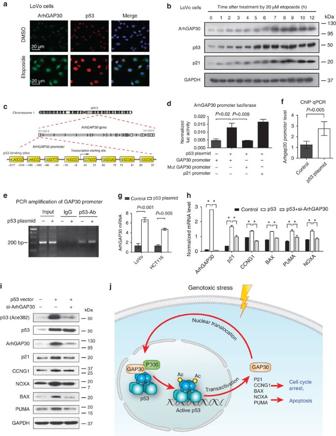Figure 7: ArhGAP30 is a direct transcriptional target of p53. (a) Immunofluorescence showing the upregulation and nuclear accumulation of p53 (labelled in red) and ArhGAP30 (green) in LoVo cells 24 h after exposure to etoposide. Scale bars, 20 μm. (b) Western blot detection of ArhGAP30, p21 and p53 expression at the indicated time points after treatment by etoposide. (c) Located at 1q23.2, the ArhGAP30 promoter contains multiple p53-binding sites that span from −217 to +97 in relation to the TSS (predicted binding sites labelled in yellow). (d) The luciferase reporter assay suggested that p53 can transactivate the ArhGAP30 promoter (−217 to +97) but not the mutant sequence devoid of the putative binding sites. Luciferase activity is indicated by the ratio of firefly (reporter) to renilla (normalization) signals. Error bars indicate means±s.d. (Student’st-test.n=4). (e) ChIP assay showing the binding of p53 to ArhGAP30 promoterin vivo. The p53 protein was pulled down in LoVo cells, and specific primers were used to amplify the ArhGAP30 promoter in the recovered DNA from the IP complex. (f) ChIP coupled to qPCR (ChIP qPCR) revealed that ectopically expressed p53 could also bind to the promoter of ArhGAP30in vivo. Error bars indicate means±s.d. (Studentt-test.n=4). (g) p53 transactivated ArhGAP30 in CRC cells. The LoVo and HCT116 cells were transfected with p53, and detected for the level of ArhGAP30 by qRT–PCR. Data represent means±s.d. (P<0.001 and 0.005, respectively, Student’st-test.n=4). (h) qRT–PCR assay showing the expression ofp21, CCNG1, BAX, PUMA, NOXAandArhGAP30genes in cells that were transfected with p53 with or without specific siRNAs for ArhGAP30. Results were based on four independent experiments (*P<0.01, Student’st-test, error bars indicate means±s.d.). (i) Western blot analysis on the expression of Ace-p53, total p53, ArhGAP30, p21, CCNG1, NOXA, BAX and PUMA proteins in the cells described above. (j) The proposed ArhGAP30-dependent mechanism for p53 functional activation. In response to DNA damage stress, ArhGAP30 is enriched in the cell nucleus. There, it binds both p53 and P300, promoting the acetylation of p53 Lys382 by P300. This activates p53 protein and facilitates the expression of downstream genes that are involved in cell cycle arrest and apoptosis. ArhGAP30 is also a direct transcriptional target of p53, thereby constituting a positive feedback circuit for p53 activation. Figure 7: ArhGAP30 is a direct transcriptional target of p53. ( a ) Immunofluorescence showing the upregulation and nuclear accumulation of p53 (labelled in red) and ArhGAP30 (green) in LoVo cells 24 h after exposure to etoposide. Scale bars, 20 μm. ( b ) Western blot detection of ArhGAP30, p21 and p53 expression at the indicated time points after treatment by etoposide. ( c ) Located at 1q23.2, the ArhGAP30 promoter contains multiple p53-binding sites that span from −217 to +97 in relation to the TSS (predicted binding sites labelled in yellow). ( d ) The luciferase reporter assay suggested that p53 can transactivate the ArhGAP30 promoter (−217 to +97) but not the mutant sequence devoid of the putative binding sites. Luciferase activity is indicated by the ratio of firefly (reporter) to renilla (normalization) signals. Error bars indicate means±s.d. (Student’s t -test. n =4). ( e ) ChIP assay showing the binding of p53 to ArhGAP30 promoter in vivo . The p53 protein was pulled down in LoVo cells, and specific primers were used to amplify the ArhGAP30 promoter in the recovered DNA from the IP complex. ( f ) ChIP coupled to qPCR (ChIP qPCR) revealed that ectopically expressed p53 could also bind to the promoter of ArhGAP30 in vivo . Error bars indicate means±s.d. (Student t -test. n =4). ( g ) p53 transactivated ArhGAP30 in CRC cells. The LoVo and HCT116 cells were transfected with p53, and detected for the level of ArhGAP30 by qRT–PCR. Data represent means±s.d. ( P <0.001 and 0.005, respectively, Student’s t -test. n =4). ( h ) qRT–PCR assay showing the expression of p21, CCNG1, BAX, PUMA, NOXA and ArhGAP30 genes in cells that were transfected with p53 with or without specific siRNAs for ArhGAP30. Results were based on four independent experiments (* P <0.01, Student’s t -test, error bars indicate means±s.d.). ( i ) Western blot analysis on the expression of Ace-p53, total p53, ArhGAP30, p21, CCNG1, NOXA, BAX and PUMA proteins in the cells described above. ( j ) The proposed ArhGAP30-dependent mechanism for p53 functional activation. In response to DNA damage stress, ArhGAP30 is enriched in the cell nucleus. There, it binds both p53 and P300, promoting the acetylation of p53 Lys382 by P300. This activates p53 protein and facilitates the expression of downstream genes that are involved in cell cycle arrest and apoptosis. ArhGAP30 is also a direct transcriptional target of p53, thereby constituting a positive feedback circuit for p53 activation. Full size image Although ArhGAP30 can be transactivated by p53, we have not found a strong correlation between the expression of ArhGAP30 and p53 in CRC tissues ( Supplementary Fig. 7b ). Also, ArhGAP30 expression level was not significantly higher in tumours carrying WT p53 ( Supplementary Fig. 7c ). These finding suggests that ArhGAP30 may also be regulated by other unknown genes in CRC (supported by different putative transcription factor binding sites on the promoter). By analysing published microarray data, we found that ArhGAP30 is significantly downregulated in prostate cancer and pancreatic cancer as compared with normal tissues ( Supplementary Fig. 7d,e ). Since BRD7 has also been found to affect p53 acetylation and function [44] , we analysed the correlation between the expression of ArhGAP30 and BRD7 in CRC tissues using The Cancer Genomic Atlas data, which revealed no significant relationship ( Supplementary Fig. 7f ). Although acetylation has been found to be crucial for p53 activation, the factors that control p53 acetylation in different physiological/pathological status are largely unclear. The findings described here implicate ArhGAP30 as a key regulator for p53 acetylation and activation in CRC. When CRC cells are exposed to DNA damage stress, ArhGAP30 is enriched in cell nucleus, where it promotes the acetylation of p53 K382 residue by p300 (schematic representation in Fig. 7j ). This modification induces p53 activation and facilitates the transcription of downstream target genes involved in cell cycle arrest and apoptosis. The colorectal epithelium is under a strong mutagenic environment [49] , thus mutated cells must be properly removed. The abundant expression of ArhGAP30 may allow readily activation of p53 function and removal of damaged cells. The effect on p53 acetylation appeared to be highly specific for ArhGAP30 full-length isoform, since the shorter variant lacking the Glu-rich domain was found without such effect. Similarly, other members of RhoGAP family that do not contain such Glu-rich domain were not regulators for p53 acetylation. These findings support the important roles of ArhGAP30 in p53 acetylation and activation in CRC. Acetylation of p53 K382 by p300 has been found to promote p53 activation, and recent studies have identified a new class of ‘bridge’ molecules that promote the binding of p300 to p53, including BRD7 (ref. 44 ), PNR/NR2E3 (ref. 50 ), WTX [37] and RUNX1 (ref. 51 ). Interestingly, the pro-p53 effects are often independent of the canonical activities of these proteins. In support of these findings, our data demonstrate that ArhGAP30 promotes p53 K382 acetylation by p300 even when the PRD of p53 (a known p300-interacting region) is completely removed. Thus, ArhGAP30 also seems to act as a bridge molecule that facilitates p300 to bind and to acetylate p53. By testing the effects of the GAP-deficient mutant of ArhGAP30, we found that ArhGAP30’s effects on p53 acetylation and function are independent of its activities as a RhoGAP. The R55A mutant, although without the ability to regulate Rho GTPase, could still promote the transactivation of p53 target genes in a p53-dependent manner, leading to suppressed cell growth, migration and increased cell apoptosis. These findings suggest significant Rho-independent but p53-dependent functions of ArhGAP30, which may link to its Glu-rich domain. In fact, many RhoGAPs contain multiple domains, some of which have unknown structures and functions. Our findings suggest the importance of characterizing the functions of these domains. The prognostic power of ArhGAP30 for CRC has been supported by both our data and the independent validation set. The association between ArhGAP30 downregulation and shorter patient survival remained significant after adjustment for AJCC stage, sex, age and microsatellite instability status. Of note, the prognostic effect of ArhGAP30 seemed to be much stronger in CRCs carrying WT p53, which is consistent with its p53-dependent tumour suppressor functions. In future clinical studies, ArhGAP30 may be used as a co-factor for p53 gene status when predicting the outcome of cancers. Finally, the potential therapeutic value for rescuing ArhGAP30 expression was demonstrated by the in vivo xenograft study, wherein ectopic expression of ArhGAP30 induced p53 activation and efficiently suppressed tumour growth. In our previous study, we have identified a ‘bridge’ molecule (synbindin) that binds ERK protein to facilitate its phosphorylation by MEK (PTM that activates ERK), and the upregulation of synbindin promotes the activation of ERK/MAPK oncogenic signalling and associates with poor survival of gastric cancer patients [52] . Although such ‘bridge’ molecules do not directly execute the PTM of the signalling protein, they can affect the extent of PTM by recruiting the enzyme to the substrate protein. Therefore, the expression of such ‘bridge’ molecule may affect cancer phenotype and serve as prognostic or therapeutic factors. In future studies, it is worth to investigate whether such bridge molecules may represent a more widespread mechanism for the regulation of cancer-related signalling. In conclusion, this study identifies ArhGAP30 as a key regulator for p53 acetylation, and suggests ArhGAP30 as both prognostic marker and potential therapeutic target for CRC. Patients and CRC biopsy specimens A total of 50 pathologically confirmed CRC patients were enrolled and underwent surgery at Renji Hospital, affiliated to the Shanghai Jiaotong University School of Medicine, between January 2005 and December 2005. The study was approved by the ethics committee of Shanghai Jiao Tong University School of Medicine, and written informed consent was obtained from all patients at study entry. Both CRC and paired normal tissues (taken at least 5 cm from the tumour were confirmed to be normal by histological examination) were analysed for ArhGAP30 protein expression by immunofluorescence, and 18 cases were analysed for ArhGAP30 mRNA level by RT–qPCR. Two tissue microarrays including 180 pairs of CRC and corresponding non-tumour tissues are purchased from BioChip (Shanghai, China), of which 169 cases detected by immunofluorescence were with survival information and included in univariate and multivariate survival analyses. The immunofluorescence assay (comparing ArhGAP30 expression in normal and CRC tissues) was based on 50 cases from Renji hospital and 180 cases from tissue microarray (in Fig. 1b ), and the analysis of clinicopathological features excluded a few cases because of missing data (in Supplementary Table 1 ). Plasmids construction The pcDNA3-HA-p53 was constructed by inserting PCR-amplified cDNA sequences into pcDNA3 vector (Invitrogen). The expression vectors pCMV6-Flag-ArhGAP30 are commercially available (OriGene). The transcriptional activity of p53 was examined by PG13-luciferase reporter plasmid that contains 13 contiguous p53 DNA-binding sites upstream of the firefly luciferase gene. The pRL-CMV vector (Promega), carrying a Renilla luciferase was used as a control vector. For ArhGAP30 luciferase assay, the promoter of ArhGAP30 (−217 to 97 in relation to TSS) was cloned and inserted into pGL3 vector. The mutant promoter (devoid of the predicted binding sites) was generated by DNA synthesis and inserted into pGL3 vector as control. Gene expressing profiling To measure relative expression of mRNA transcripts, tissue RNA samples were analysed using Affymetrix HG U133 Plus 2.0 GeneChips (Affymetrix, Santa Clara, CA) according to the manufacturer’s protocols. Biotin-labelled cRNA was prepared using 5 μg (1.0 μg μl −1 ) total RNA (1 μg mRNA) with the ‘One-Cycle cDNA’ kit (incorporating a T7-oligo (dT) primer) and the GeneChip IVT labelling kit. In vitro transcribed cRNA was fragmented (20 μg) and analysed for quality control purposes by spectrophotometry and gel electrophoresis before hybridization. Finally, a hybridization cocktail was prepared with 15 μg of cRNA (0.5 μg μl −1 ) and hybridized to HG U133 Plus 2.0 microarrays for 16 h at 45 °C in an Affymetrix Hybridization Chamber 640. Each cRNA sample was spiked with standard prokaryotic hybridization controls for quality monitoring. Hybridized microarrays were stained with streptavidin phycoerythrin and washed with a solution containing biotinylated anti-streptavidin antibodies using the Affymetrix Fluidics Station 450. Finally, the stained and washed microarrays were scanned with the Affymetrix Scanner 3000. The Affymetrix software package was used to transform raw microarray image files to digitized format. As for the Discovery set above, gene expression levels for the validation data set were calculated using MAS 5.0 (Affymetrix) for quality control purposes and with the RMA normalization algorithm for expression data. The pathways associated with ArhGAP30-upregulated genes (criteria: P <0.05, t -test, fold change >1.5) were analysed by Gene Ontology annotation using the DAVID tool [53] with default parameters of the algorithm. ChIP assay The ChIP assays were performed using a ChIP kit (Millipore), according to the manufacturer’s instructions. Briefly, 1 × 10 7 cells and 5 μg anti-p53 antibody were used for each ChIP experiment. Mouse immunoglobulin G was used as a negative control. An iCycler iQ real-time PCR detection system (Bio-Rad) was used to perform the qPCR. The DNA sequence surrounding the p53-binding site in the human ArhGAP30 promoter was amplified from immunoprecipitated protein–DNA complexes using the following primer pair: forward 5′-CAAGCAAAGGGTGAGGATGT-3′, reverse 5′-GTGGCTGTTGAAGAGGAAGC-3′. The primers for amplifying other p53 targets are as following (forward and reverse sequences for each gene): CDKN1A 5′-AGCAGGCTGTGGCTCTGATT-3′, 5′-CAAAATAGCCACCAGCCTCTTCT-3′;CCNG1 5′-ACCTCCTGCCTTCCTGTCTTTA-3′, 5′-GCACAAGCTAAGCCCTGGAT-3′; BAX 5′-CGCTCTCGGACCCTCGAGAA-3′, 5′-TGCATCCAGACCCCTGGCCT-3′; PUMA 5′-TGTCCATGGTGTGGATTTGCG-3′, 5′-AGACACCGGGACAGTCGGACA-3′ NOXA 5′-CAGCGTTTGCAGATGGTCAA-3′, 5′-CCCCGAAATTACTTCCTTACAAAA-3′. ChIP-seq data analysis The p53 ChIP-seq data are obtained from a published study, and the raw reads were downloaded from GEO database (GSE46641). All sequence reads generated from Illumina Genome Analyzer II were aligned against human reference sequence (GRCh37p5, or hg19, June 2011) using Burrows-Wheeler Alignment tool [54] . The uniquely mapped short reads were used to identify regions of the genome with significant enrichment in p53-associated DNA sequences. The peak detection was performed by QuEST 2.4 software [55] using the ‘Transcription factor binding site’ setting (bandwidth of 30 bp, region size of 300 bp) and the ‘stringent peak calling’ parameters (corresponding to 50-fold ChIP to input enrichment for seeding the regions and threefold ChIP enrichment for extending the regions). The p53-binding regions (p53BR) were analysed for their distances to the TSSs of ArhGAP30-upregulated genes using the ChIPpeakAnno tool [56] with default parameters of the algorithm. In vivo experiments Briefly, male BALB/c athymic nude mice (4–5 weeks old) were obtained from the Experimental Animal Center of SIBS. Mice were randomly divided into two groups (eight mice per group): control and ArhGAP30 group. Control group mice were injected subcutaneously into the right armpit with 1.0 × 10 7 LoVo cells bearing empty plasmid vector, whereas the ArhGAP30 group mice were injected with 1.0 × 10 7 LoVo cells bearing ArhGAP30 plasmid to establish a CRC xenograft model. Tumour diameters were measured at regular intervals with digital calipers, and tumour volume was calculated by the formula: tumour volume (mm 3 )=0.5 × shorter diameter 2 × longer diameter 2 . The tumour volume data are presented as means±s.d. ( n =8). After 3 weeks, all mice were killed and subcutaneous tumours were collected for analysis. Our study was approved by the Animal Care and Use Committee of the Shanghai Jiao-Tong University School of Medicine Renji Hospital, Shanghai, China. All animal procedures were performed according to the guidelines developed by the China Council on Animal Care, and the protocol was approved by the Shanghai Jiao-Tong University School of Medicine, Renji Hospital, Shanghai, China. Statistical analysis Data are presented as the mean±s.d. Comparisons were performed using the Student’s paired t -test, Spearman’s correlation test, or χ 2 -test. P <0.05 was considered as statistically significant. Accession codes: Microarray data have been deposited in the Gene Expression Omnibus database under accession code GSE49536 . How to cite this article : Wang, J. et al. ArhGAP30 promotes p53 acetylation and function in colorectal cancer. Nat. Commun. 5:4735 doi: 10.1038/ncomms5735 (2014).